Interplay between Notch1 and Notch3 promotes EMT and tumor initiation in squamous cell carcinoma Notch1 transactivates Notch3 to drive terminal differentiation in stratified squamous epithelia. Notch1 and other Notch receptor paralogs cooperate to act as a tumor suppressor in squamous cell carcinomas (SCCs). However, Notch1 can be stochastically activated to promote carcinogenesis in murine models of SCC. Activated form of Notch1 promotes xenograft tumor growth when expressed ectopically. Here, we demonstrate that Notch1 activation and epithelial–mesenchymal transition (EMT) are coupled to promote SCC tumor initiation in concert with transforming growth factor (TGF)-β present in the tumor microenvironment. We find that TGFβ activates the transcription factor ZEB1 to repress Notch3 , thereby limiting terminal differentiation. Concurrently, TGFβ drives Notch1-mediated EMT to generate tumor initiating cells characterized by high CD44 expression. Moreover, Notch1 is activated in a small subset of SCC cells at the invasive tumor front and predicts for poor prognosis of esophageal SCC, shedding light upon the tumor promoting oncogenic aspect of Notch1 in SCC. Notch signaling regulates cell fate in a context-dependent manner [1] . The ligand-activated intracellular domain of Notch (ICN) forms a transcriptional activation complex with the transcription factor CSL and the co-activator MAML. Notch1 drives terminal differentiation in stratified squamous epithelia [2] , [3] in concert with other Notch receptor paralogs [4] , [5] . Histopathology of squamous cell carcinomas (SCCs) features squamous-cell differentiation, a process normally regulated via direct transcriptional activation of Notch3 by ICN1, the activated form of Notch1, in esophageal epithelia [4] . Loss-of-function Notch1 mutations are found in SCCs [6] , [7] , suggesting a tumor suppressor role for Notch1 [5] , [8] , [9] . However, Notch1 can be stochastically activated or inactivated, with either scenario resulting in promotion of carcinogenesis in murine models of SCC [10] . Many human SCC cell lines express ICN1 and ectopic ICN1 expression promotes xenograft tumor growth [11] , [12] . While pharmacological modulation of Notch paralogs represents an attractive strategy for cancer therapy [13] , a more detailed understanding of the functional role of the Notch pathway as it relates to tissue biology in the context of health and disease is necessary to guide such approaches. In addition to squamous-cell differentiation, Notch1 regulates cell cycle [3] , [12] , [14] , senescence [12] , and epithelial–mesenchymal transition (EMT) [15] , [16] , [17] . Acquisition of mesenchymal properties facilitates malignant transformation by limiting oncogene-induced senescence [18] , [19] . In human esophageal squamous cell carcinoma (ESCC), the deadliest form of all human SCCs [20] , EMT is associated with chemoresistance and poor prognosis [21] , [22] , [23] . EMT also regulates cancer stem cells (CSCs) [24] , [25] . CSCs defined by high CD44 expression (CD44H) have been identified in various tumor types, including SCCs [26] , [27] , [28] , [29] . In transformed esophageal and oral keratinocytes, cells with low CD44 expression (CD44L) and epithelial properties are converted to CD44H cells with mesenchymal traits in response to transforming growth factor (TGF)-β [30] , [31] , a potent EMT inducer present in the tumor microenvironment [32] . During TGFβ-mediated EMT, expression of the Notch ligand JAG1 is induced via ZEB1 [12] , [15] , [33] , a transcription factor essential in TGFβ-induced EMT [34] , [35] and microRNA-mediated regulation of Notch signaling [33] , [36] , [37] . While emerging lines of evidence support Notch1 as a positive effector of EMT [15] , [16] , [17] , [37] , [38] , Notch3 limits the expansion of EMT-competent esophageal keratinocytes [11] . Thus, although Notch1 and Notch3 cooperate to drive squamous-cell differentiation [4] , these Notch paralogs may play opposing roles in EMT and, potentially, regulation of CSC dynamics. The precise molecular mechanisms through which Notch signaling regulates distinct cell fates in a context-dependent manner have yet to fully elucidated. Here, we aimed to define the functional role of Notch1 in SCC. We demonstrate that Notch1 activation and EMT are coupled to promote tumor initiation and intratumoral cancer cell heterogeneity in SCC. We find that the transcription factor ZEB1 represses NOTCH3 , thereby limiting ICN1-induced differentiation while permitting ICN1-mediated EMT. Moreover, ICN1 expression in a small subset of SCC cells at the invasive tumor front predicts independently for poor prognosis of ESCC. These findings suggest an oncogenic role for Notch1 in SCC and identify the TGFβ–ZEB1–Notch1 axis as potential target for SCC therapy. EMT and Notch1 activation are features of carcinogen-driven ESCC in vivo To study SCC initiation and progression in vivo, we treated mice with 4-Nitroquinoline 1-oxide (4NQO), a potent oral-esophageal carcinogen. We combined 4NQO treatment with a cell-lineage tracing experimental system in which murine oral and esophageal epithelial basal cells (keratinocytes) were marked permanently with tdTomato fluorescent protein following tamoxifen (TAM)-induced Cre-mediated recombination in K5Cre ERT2 ;R26tdTomato lsl/lsl mice (Fig. 1a ). 4NQO-induced lesions showed tdTomato accumulation (Fig. 1b ; Supplementary Fig. 1a, b ), validating the basal keratinocyte origin of these tumors [39] . Flow cytometry revealed the presence of cells displaying both negative and positive expression of EpCAM (EpCAM neg and EpCAM pos ), an epithelial cell surface marker, within the tdTomato-positive (tdTomato pos ) fractions of 4NQO-induced ESCC lesions (Supplementary Fig. 1c ), suggesting a loss of epithelial characteristics in tumor cells originating from esophageal basal keratinocytes. In cell lineage tracing experiments, tdTomato expression assures that these EpCAM neg cells are not co-existing intratumoral stromal cells (e.g., fibroblasts) which are not labeled with tdTomato via K5Cre ERT2 . Quantitative reverse-transcription polymerase chain reaction (qRT-PCR) analysis coupled with fluorescence-activated cell sorting (FACS) demonstrated further upregulation of genes associated with mesenchymal cells (Fig. 1c ) including Zeb1 , in tdTomato pos ;EpCAM neg cells originating from basal esophageal keratinocytes. Consistent with EMT as described in human ESCC [11] , neoplastic lesions displayed E-cadherin loss or mislocalization as well as robust Zeb1 expression at the stromal interface (Fig. 1d ). Single-cell-derived three-dimensional (3D) organoids generated from 4NQO-induced dysplastic mucosa and primary tumors recapitulated acquisition of mesenchymal properties as found in 4NQO-induced neoplastic lesions (Fig. 1e ). We also included mice with conditional loss or expression of mutant p53 since p53 dysfunction promotes EMT [19] , [31] , [40] and found that more pronounced E-cadherin loss and reciprocal Zeb1 upregulation were observed in invasive tumors with mutant p53 R172H (Supplementary Fig. 1d ). Fig. 1 Lineage tracing reveals mesenchymal traits and Notch1 activation in ESCC lesions. a Schematic of cell-lineage tracing experiments. b Macroscopic and fluorescent images of representative tdTomato-labeled esophagus bearing 4NQO-induced tumors (arrows). Scale bar, 1 mm. c qRT-PCR analysis for indicated genes comparing EpCAM neg to EpCAM pos cells from a representative tdTomato-labeled tumor. * P < 0.0001 and # P < 0.05 vs. EpCAM pos , n = 3. d Representative IF images for Zeb1 and E-cadherin (E-cad) in normal mucosa (top) and ESCC (bottom). Dashed line denotes interface between stroma and basal keratinocytes (top) or invasive ESCC cells (bottom). Note E-cadherin downregulation in ESCC cells with nuclear Zeb1 (arrowheads) at the tumor invasive front. Scale bar, 50 µm. e H&E, multicolor IF for E-cadherin and Zeb1, and IHC for ICN1 (ICN1 Val1744 ) in representative single-cell-derived organoids from normal mucosa or 4NQO-induced tumors. Note that spherical organoids from 4NQO-untreated control mice exhibit a differentiation gradient with predominant luminal keratinization, whereas tumor-derived organoids (neoplastic) display irregular morphology with increased cellularity and diminished keratinization. Zeb1 expression was robust in tumor organoids, particularly at invasive protrusions with decreased E-cadherin expression and detectable ICN1 expression. Box denotes area magnified in panel below. Scale bars, 20 µm. f Representative IHC image for ICN1 4NQO-induced IEN (dysplasia) containing spindle-shaped cells (arrowheads). Scale bar, 50 µm. g Quantification of ICN1 IHC scoring in normal mucosa and 4NQO-induced lesions in mice of indicated genotype. * P < 0.05 vs. p53 +/+ ( K5Cre ERT2 ;R26tdTomato lsl/lsl ) normal, # P < 0.0005 vs. p53 −/− ( K5Cre ERT2 ;R26tdTomato lsl/lsl ; p53 loxP/loxP ) normal; † P < 0.05 vs. p53 −/− IEN; ns not significant vs. p53 +/+ normal. Data in b – f represent at least three independent 4NQO-induced lesions and >20 organoids from at least two independent experimental replicates. In g , n = 5 normal, n = 8 IEN, and n = 5 invasive ESCC in p53 +/+ esophagi. N.D. not detectable. n = 3 normal, n = 7 IEN, n = 5 invasive ESCC, and n = 4 metastatic tumors in p53 −/− esophagi. Two independent experimental replicates were carried out. Bar diagrams represent mean ± s.d. in c and mean ± s.e.m. in g . Student’s t -test was used for paired data comparisons in c , g . ANOVA with Tukey’s post hoc test was used for multiple comparisons in g Full size image We next utilized this experimental platform to examine expression of ICN1 (ICN1 Val1744 ), the activated form of Notch1, throughout the natural history of ESCC. In comparison to normal esophageal squamous epithelia, ICN1 expression was increased in dysplastic lesions and remained upregulated in primary and metastatic ESCC (Fig. 1f, g ; Supplementary Fig. 1e ). Moreover, ICN1 was detected in invasive ESCC cells displaying E-cadherin mislocalization and Zeb1 upregulation (Supplementary Fig. 1d ). ICN1 was also expressed highly in neoplastic organoids displaying EMT (Fig. 1e ), suggesting a potential role for ICN1 in the acquisition of mesenchymal properties by SCC cells. The tumor suppressor p53 protein can transcriptionally activate Notch1 in response to genotoxic stress [41] . Since 4NQO activates p53 via DNA damage [42] , ICN1 expression in 4NQO-induced early lesions may reflect p53 activation in dysplastic cells. Conversely, Notch1 downregulation may be accounted for by p53 inactivation during disease progression. Therefore, we evaluated the influence of p53 loss upon ICN1 expression in the esophageal epithelium. TAM-induced K5Cre ERT2 -driven p53 loss did not affect ICN1 expression in mice without 4NQO treatment ( P = 0.06 by Student’s t -test; n = 3 animals per group; two independent experimental replicates), a finding that recapitulates p53 −/− murine epidermis [43] . When p53 was deleted in oral-esophageal keratinocytes then mice were treated with 4NQO, p53 loss did not prevent ICN1 expression in neither normal esophageal epithelium nor 4NQO-induced neoplastic lesions (Fig. 1g ; Supplementary Fig. 1e ). Mice with p53 deletion did, however, display frequent metastases (Supplementary Fig. 1a ). These findings suggest that p53 may be dispensable for Notch1 activation in 4NQO-induced lesions, albeit essential for overall SCC progression. Notch1 promotes ESCC tumorigenicity and expansion of CD44H cells with mesenchymal properties To explore further the functional role of Notch1 in ESCC tumorigenicity, we first utilized the extensively characterized human ESCC cell lines TE11 and EN60 [12] . Both express ICN1 and form tumors upon xenograft transplantation in immunodeficient mice where doxycycline (DOX)-inducible ectopic ICN1 augments tumor growth [11] , [12] . To assess Notch activity in vivo, we used 8×CSL-GFP , a lentiviral green fluorescent protein (GFP) reporter driven by the minimal SV40 promoter fused to concatemeric CSL-binding sites (Fig. 2a ). In TE11 and EN60 xenograft tumors, a subset of turboRFP (tRFP)-expressing tumor cells exhibited CSL-mediated transcriptional activity (Fig. 2b ). A functional role for Notch activity in ESCC tumor growth is evident as dominant negative mutant MAML1 ( DNMAML1 ) [44] prevented DOX-induced ectopic ICN1 from stimulating tumor growth (Fig. 2c ). Additionally, DNMAML1 alone or NOTCH1 -directed short hairpin RNA (shRNA) suppressed tumor volume significantly (Fig. 2c, d ). CRISPR/Cas9-mediated NOTCH1 deletion dramatically impaired tumor formation by TE11 cells in immunodeficient mice (Fig. 2e ), supporting a role for Notch1 in tumor initiation as well. EN60 cells are less tumorigenic than TE11 upon xenograft transplantation, displaying 12.5–25% tumor formation rates with 1–4 × 10 6 cells transplanted; however, DOX-induced ectopic ICN1 enhanced EN60 tumor formation rate to 100% ( P < 0.01 by Fisher’s exact test; n = 12; two independent experimental replicates). Moreover, the ability of esophageal neoplastic cells to form single-cell-derived 3D organoids was attenuated upon Cre-mediated ex vivo Notch1 deletion in single-cell suspensions prepared from dysplastic lesions or ESCC tumors of 4NQO-treated Notch1 loxP/loxp mice (Fig. 2f ). Fig. 2 Notch1 promotes ESCC tumorigenesis. a Schematic of 8×CSL-GFP reporter. Notch activation permits GFP reporter expression via concatemeric CSL-binding sites. Constitutively active UBC promoter drives tRFP expression concurrently. Cells without tRFP represent host-derived stromal cells. b Representative flow cytometry scatter plots determining 8×CSL -mediated GFP reporter activation, indicating Notch active population of tRFP-labeled ESCC cells in TE11 and EN60 xenograft tumors. On average, 43.5 ± 0.5% s.d. of EN60 and 11.2 ± 6.5% s.d. of TE11 cells comprised the live GFP Pos /tRFP Pos fraction across three independent tumors. c , d Tumor growth curves in immunodeficient mice carrying TE11 tumors of indicated genotypes. Upon xenograft transplantation, mice were treated with DOX to induce ICN1 or NOTCH 1-directed shRNA. Tumor growth was monitored for indicated time periods. In c , * P < 0.01 vs. zeo and DOX (−), # P < 0.05 vs. zeo and DOX (+), n = 6–8 per group. In d , * P < 0.05 vs. DOX (−); n = 6 per group. e TE11 cells with CRISPR/Cas9-mediated NOTCH1 deletion. Immunoblotting confirms ICN1 loss in NOTCH1 -deleted TE11 (N1 Δ ), but not non-targeted control TE11 (N1 WT ) cells. Bar graph shows tumor formation rate in immunodeficient mice 7 weeks after xenograft transplantation. * P < 0.05 vs. N1 WT , n = 8 per group. f Esophageal keratinocytes isolated from 4NQO-induced IEN (dysplasia) lesions or ESCC tumors of Notch1 loxP/loxP mice were utilized to generate 3D esophageal organoids in the presence or absence of ex vivo Cre-mediated recombination. qRT-PCR analysis confirms inhibition of Notch1 gene expression upon ex vivo Cre-mediated recombination in ESCC organoids. * P < 0.000 vs. Cre (−), n = 3. Organoid formation rate was evaluated at day 14 post-plating and is represented as relative to Cre (−) for IEN and ESCC. * P < 0.000 vs. Cre (−) IEN; # P < 0.001 vs. Cre (−) ESCC. Line graphs represent mean ± s.e.m. in c , d . Bar diagrams represent mean ± s.d. in f . At least two independent replicates were performed for all experiments. Repeated measures ANOVA with Tukey’s post hoc test were used for multiple comparisons in c , d . Chi square with Fisher’s exact test was used for percentage comparisons in e . Student’s t -test was used for paired data comparisons in f Full size image Human SCC tumors comprise CD44L and CD44H cells, the latter exhibiting augmented tumor-initiating capability [28] , [29] . CD44H expression is associated with mesenchymal characteristics in transformed oral-esophageal cell lines [31] . Following FACS-purification, early passage CD44H TE11 and EN60 cells maintained enhanced expression of the mesenchymal cell marker N-cadherin as compared to their CD44L counterparts in culture (Supplementary Fig. 2a ). Additionally, CD44H cells isolated from TE11 and EN60 xenograft tumors exhibited upregulation of ZEB1 and CDH2 (N-cadherin) (Fig. 3a ; Supplementary Fig. 2b ). As ectopic ICN1 expression in EN60 tumors enhanced robustly intratumoral CD44H cell content (Fig. 3b ), we hypothesized that Notch1 contributes to tumor initiation via generation of CD44H cells that have mesenchymal properties. To determine how Notch1 may influence tumor initiation by CD44L and CD44H cells, we performed serial transplantation experiments (Fig. 3c ). We first grew tumors without activating DOX-inducible ICN1. We then purified CD44L and CD44H cells by FACS from primary tumors and 1 × 10 3 cells were serially injected into recipient mice where DOX was given to induce ectopic ICN1 expression. CD44L cells purified from EN60 and TE11 tumors showed low (<30%) spontaneous tumor formation efficiency; however, ICN1 dramatically stimulated tumor initiation by CD44L cells to 80–90%. In TE11 CD44L cells, DNMAML1 not only antagonized ICN1-mediated tumorigenicity, but also suppressed spontaneous tumor formation. While purified CD44H cells were highly tumorigenic (80–100%), neither ectopic ICN1 nor DNMAML1 affected tumor initiation by CD44H cells, suggesting that established CD44H-mediated tumor initiation is independent of Notch1. To our knowledge, this is the first demonstration that Notch1 may facilitate tumor initiation by converting CD44L cells to highly tumorigenic CD44H cells with mesenchymal traits in vivo. Fig. 3 Notch1 facilitates expansion of CD44H cells with mesenchymal properties. a qRT-PCR analysis for indicated genes comparing EN60 intratumoral CD44L and CD44H cells. * P < 0.05 vs. CD44L; # P < 0.0001 vs. CD44L; n = 3 per group. b Representative flow cytometry scatter plot determining CD44H cells in EN60 tumors grown for 4 weeks with or without DOX-induced ICN1 (EN60- ICN1 TetOn ). c Experimental design of serial transplantation experiments and tumor formation rates by CD44L and CD44H cells purified from parental xenograft tumors carrying DOX-inducible ICN1 (EN60- ICN1 TetOn and TE11- ICN1 TetOn ). Parental tumors were grown in mice without DOX treatment and dissociated for FACS-purification of CD44L and CD44H cells. Purified cells were serially transplanted (10 3 cells per injection site) into recipient mice to monitor tumor formation. Recipient mice were treated with or without DOX. TE11 carried DNMAML1 or zeo (empty vector control). * P < 0.05 for CD44L and DOX (+) vs. CD44L and DOX (−), n = 10–12 per group; ns not significant for CD44L and DOX (+) vs. CD44H (with or without DOX treatment), n = 10 per group; # P < 0.05 vs. TE11- ICN1 TetOn -zeo CD44L and DOX (+), n = 10 per group. d Flow cytometry analysis for EpCAM-negative cells in TE11 with NOTCH1 deletion (N1 Δ ) or wild-type control (N1 WT ). Cells were treated with or without 5 ng/ml TGFβ for 72 h. * P < 0.05 vs. TGFβ (−); # P < 0.0001 vs. N1 WT and TGFβ (+), n = 3. Data are presented as mean ± s.e.m. e Multicolor IF for E-cadherin and Zeb1 in representative single-cell-derived organoids from 4NQO-induced ESCC tumors of Notch1 loxP/loxP mice with or without ex vivo Cre-mediated recombination. Zeb1 expression diminished in organoids upon Cre-mediated Notch1 deletion (arrowheads). Box denotes area that is magnified in panel below. KC keratinized core of organoids. Scale bars, 20 µm. Bar diagrams represent mean ± s.d. in a , d . At least two independent replicates were performed for all experiments. Student’s t -test was used for paired data comparisons in a , d . Chi square with Fisher’s exact test was used for percentage comparisons in c Full size image TGFβ and Notch1 cooperate to drive EMT in the tumor microenvironment The functional role of Notch1 in EMT was suggested as NOTCH1 deletion in cultured TE11 cells attenuated sharply TGFβ-mediated EpCAM neg cell induction (Fig. 3d ). Cre-mediated ex vivo Notch1 deletion in 3D ESCC organoids generated from 4NQO-induced Notch1 loxP/loxP murine tumors resulted in a diminished expression of Zeb1 (Fig. 3e ). Moreover, DOX-induced ectopic ICN1 augmented intratumoral EpCAM neg cell content in TE11 xenograft tumors (Supplementary Fig. 2c ). While these data support a role for Notch1 in promotion of ESCC tumor cells with attributes of EMT, EpCAM neg cells were rare in cultured TE11 cells and ectopic ICN1 expression alone had no influence upon this cell population (Supplementary Fig. 2c ), indicating that Notch1 activation alone may not be sufficient to drive EMT. In the tumor microenvironment, Notch signaling may be modulated by other transcription factors such as HIF1α [17] and SMAD3 [45] via physical interactions with ICN1. We suspected that TGFβ influences Notch1-mediated tumor promotion and EMT since the TGFβ target gene PAI1 was upregulated in CD44H cells in tumors (Fig. 3a ; Supplementary Fig. 2b ). In agreement, an anti-TGFβ blocking therapeutic monoclonal antibody 1D11 [46] severely impaired tumor growth of TE11 xenograft tumors as well as OCTT2 head and neck SCC patient-derived xenografts (PDXs) (Fig. 4a ). In the context of 4NQO-mediated carcinogenesis, the percentage of esophageal mucosa occupied by neoplastic lesions classified as intraepithelial neoplasia (IEN) or ESCC was diminished upon treatment with 1D11 (26.0% ± 8.1 s.e.m. ; n = 5) as compared to isotype control (56.3% ± 14.2 s.e.m. ; n = 4; P = 0.09 by Student’s t -test; two independent experimental replicates). Administration of 1D11 to 4NQO-treated animals further attenuated ICN1 expression as well as morphological evidence of EMT in esophageal epithelium (Fig. 4b, c ). Taken together, these data indicate that TGFβ functions as a critical positive effector of Notch1 and EMT in the context of the tumor microenvironment. Fig. 4 TGFβ signaling facilitates ESCC tumor growth, Notch1 signaling, and EMT. a Growth curve for mice bearing TE11 or HNSCC PDX tumors receiving either ID11 anti-TGFβ blocking antibody or control IgG via intraperitoneal injection at indicated time points (arrows). ID11 neutralizes all TGFβ isoforms. * P < 0.05 vs. IgG, n = 5–8 per group. b , c p53 +/+ mice were treated with 4NQO for 16 weeks. Six weeks following 4NQO withdrawal, mice were treated with ID11 anti-TGFβ blocking antibody or control IgG via intraperitoneal injection three times weekly for a period of 2 weeks. In b , quantification of ICN1 IHC scoring in esophageal epithelium with representative IHC images for IgG-treated and anti-TGFβ blocking antibody-treated animals. * P < 0.05; n = 4–5 per group. Scale bar, 50 µm. In c , multicolor IF for E-cadherin and Zeb1 in representative 4NQO-induced IEN lesions from IgG-treated and anti-TGFβ blocking antibody-treated animals. Data indicate mean ± s.e.m. in a , b . At least two independent replicates were performed for all experiments. Repeated measures ANOVA with Tukey’s post hoc test were used for multiple comparisons in a . Student’s t -test was used for paired data comparisons in b Full size image To dissect further the mechanistic role of Notch1 in the generation and maintenance of ESCC tumor cells with mesenchymal features, we utilized the genetically engineered transformed esophageal cell line EPC2T (EPC2-hTERT-EGFR-p53 R175H -cyclin D1), comprising discrete CD44L and CD44H subpopulations with epithelial and mesenchymal traits, respectively [31] (Supplementary Fig. 3a ). Under basal conditions, Notch activity, as measured using 8×CSL-GFP reporter (Fig. 2a ), was highest within a subset of intermediate transitioning cells (designated as CD44T) as compared to CD44L or CD44H cells (Fig. 5a ). In TGFβ-mediated EMT with a resulting increase in CD44T and CD44H cells, Notch activity was augmented further in the CD44T subpopulation (Fig. 5a ), indicating that Notch activity may be augmented transiently during the CD44L-to-CD44H transition. Induction of CD44H cells may be accounted for by expansion of pre-existing CD44H cells as well as conversion from CD44L cells. Following FACS purification, CD44H cells failed to display CD44L repopulation even after extended passage (Supplementary Fig. 3b ). CD44L cells that were cultured in the absence of TGFβ underwent expansion while permitting minimal CD44H cell repopulation within 5 weeks (four passages) (Supplementary Fig. 3b ); however, purified CD44L cells robustly gave rise to CD44H cells upon TGFβ stimulation (Supplementary Fig. 3c ; Fig. 5b ). A requirement for TGFβ in CD44H cell induction was suggested as pharmacological inhibition of TGFβ receptor-mediated signaling suppressed spontaneous conversion of purified CD44L cells to CD44H cells (Supplementary Fig. 3d ). A permissive role for Notch1 in CD44H cell generation via TGFβ-induced EMT was implicated further as a γ-secretase inhibitor (GSI), DNMAML1 or NOTCH1 -directed shRNA each individually attenuated TGFβ-mediated CD44H cell expansion from purified CD44L cells (Supplementary Fig. 3c ; Fig. 5b ). Ectopic ICN1 augmented CD44H cell expansion from TGFβ-stimulated purified CD44L cells where ICN1 failed to influence spontaneous CD44H cell expansion in the absence of TGFβ (Fig. 5c ). Taken together, these data indicate that Notch1 activation is required, but not sufficient, for EMT-mediated CD44H cell induction in EPC2T cells. Fig. 5 TGFβ-mediated Notch1 activation permits EMT and suppresses differentiation. a Representative flow cytometry scatter and histogram plots for 8×CSL-GFP reporter activity in indicated subpopulations of EPC2T cells treated with TGFβ or CaCl 2 for 72 h. b , c Flow cytometry determined CD44H cells induced in FACS-purified CD44L cells with indicated conditions or genotypes. Cells were treated with TGFβ or DOX for 7 days. * P < 0.0001 vs. TGFβ (−); # P < 0.005 vs. TGFβ (+) and DMSO, GFP , or non-silencing scrambled (NS) shRNA in b ; n = 3. * P < 0.05 vs. TGFβ (−) and DOX (−); ns not significant vs. TGFβ (−) and DOX (−); # P < 0.05 vs. TGFβ (+) and DOX (−) in c ; n = 3. d Representative H&E images of OTC reconstituted with CD44L or CD44H cells. Epi epithelia, Str stroma. Scale bar, 50 μm. e Representative flow cytometry scatter plots of purified CD44H cells treated with SB431542 or vehicle (control) for 14 days. SB431542 increased CD44L cell content (upper left quadrant) to 0.35 ± 0.08% as compared to 1.2 ± 0.1% s.d. in vehicle ( P < 0.0005, n = 3). f qRT-PCR analysis for indicated genes in FACS-purified CD44H cells treated with or without SB431542. mRNA level for each gene in vehicle-treated cells was set as 1. * P < 0.0005 vs. vehicle, n = 3. g Heat map of gene array results from EPC2T derivative (EPC2T- ICN1 TetOn ) treated with DOX and/or TGFβ ( n = 3 per condition). “Differentiation” genes were significantly increased (≥1.5-fold) by DOX-induced ectopic ICN1 alone, but suppressed by TGFβ ( P < 0.05 by two-way ANOVA). “EMT” genes activated by TGFβ (≥1.5-fold) were significantly augmented by ectopic ICN1 ( P < 0.05 by two-way ANOVA). h qRT-PCR analysis validates gene array results in g . mRNA level for DOX (−) and TGFβ (−) was set to 1. * P < 0.001 vs. TGFβ (−) and DOX (−); # P < 0.0001 vs. TGFβ (−) and DOX (+); ns not significant vs. TGFβ (−) and DOX (−); n = 3. All bar diagrams indicate mean ± s.d. Student’s t -test was used for paired data comparisons in e , f . At least two independent replicates were performed for all experiments. ANOVA with Tukey’s post hoc test were used for multiple comparisons in b , c , h Full size image Transcriptional repression of Notch3 via Zeb1 permits Notch1-mediated EMT As our findings indicate a role for Notch in EMT, we next sought to determine how Notch1 regulates cell fate in squamous epithelia. The 8×CSL-GFP reporter activity was unaffected in CD44T and CD44H cells upon calcium-mediated squamous-cell differentiation (Fig. 5a ) [4] . In CD44L cells, which displayed differentiation in organotypic 3D culture (OTC) when compared to invasive CD44H cells (Fig. 5d ), calcium treatment enhanced Notch activity in a subset of cells (Fig. 5a ). Thus, local environmental cues may impact Notch signaling to direct cell fate determination. In agreement with this notion, pharmacological inhibition of TGFβ signaling in purified CD44H cells induced CD44L cells with concurrent downregulation of EMT markers and NOTCH3 upregulation (Fig. 5e, f ). A trend toward increased Notch3 expression was also detected in peeled murine esophageal epithelia with 4NQO-induced neoplastic lesions following treatment with anti-TGFβ-blocking antibody 1D11 (Supplementary Fig. 3e ). Gene array analysis in EPC2T cells revealed further that ectopic ICN1 expression induced a gene expression pattern compatible with squamous-cell differentiation. However, TGFβ treatment in the context of ICN1-overexpression triggered a robust shift toward an EMT-associated gene expression signature (Fig. 5g ; Supplementary Fig. 3f ) (GSE37994, GSE37993). qRT-PCR analysis confirmed that ICN1 and TGFβ cooperate to induce expression of EMT regulators, including ZEB1 and SNAI1 , while TGFβ limited ICN1-mediated expression of NOTCH3 as well as IVL , the latter a marker of terminal differentiation (Fig. 5h ). Although the lack of discontinuous CD44L and CD44H cell populations in EN60 and TE11 prevented their isolation for long-term cell culture analyses, the role of Notch and TGFβ signaling in induction of CD44H cells and regulation of squamous-cell differentiation was recapitulated in TE11 cells (Supplementary Fig. 3g–i ). We investigated next the mechanistic role of Notch3 in EMT in the context of ESCC. TE11 serial transplantation experiments revealed that DOX-induced ectopic ICN3 suppressed tumor initiation by CD44L cells (Fig. 6a ). In EPC2T cells, ectopic ICN3 induced IVL in the presence or absence of TGFβ stimulation (Supplementary Fig. 4a, b ). Moreover, ectopic ICN3 abrogated TGFβ-mediated CD44H cell expansion in EPC2T cells (Supplementary Fig. 4c ), while NOTCH3 knockdown was sufficient to promote CD44H cell expansion (Fig. 6b ) coupled with decreased differentiation and increased EMT characteristics (Fig. 6c ) in the absence of TGFβ stimulation. These findings indicate that Notch3, unlike Notch1, may limit EMT so as to permit squamous-cell differentiation. To define the mechanism through which Notch3 expression is suppressed during EMT, we analyzed the NOTCH3 locus by the ECR browser [47] . This analysis predicts two conserved ZEB-binding sites in the NOTCH3 second intron ( N3Int2 ) adjacent to the CSL-binding sites (Fig. 6d ) that is occupied by ICN1 during squamous-cell differentiation [4] . Hypothesizing that ZEB transcription factors repress Notch3 , we evaluated the influence of ectopic ZEB1 or ZEB2 expression upon N3Int2 -modulated transcriptional activity. ZEB1 specifically suppressed basal pGL3-N3Int2-luc reporter activity and also abrogated reporter activation via DOX-induced ectopic ICN1 (Fig. 6e ; Supplementary Fig. 4d ). Chromatin immunoprecipitation (ChIP) analysis revealed enrichment of ZEB1 binding to the N3Int2 region in purified CD44L cells with TGFβ stimulation and purified CD44H cells without TGFβ stimulation (Fig. 6f ). TGFβ did not prevent ICN1 from binding to the N3Int2 region (Supplementary Fig. 4e ), suggesting that ZEB1 binding may predominate over ICN1 to repress NOTCH3 transcription. ZEB1 -directed shRNA attenuated TGFβ-induced CD44H cell expansion, further implicating ZEB1 as a critical positive regulator in EMT-mediated generation of CD44H cells (Fig. 6g ). Fig. 6 ZEB1 represses NOTCH3 , facilitating EMT and tumor initiation. a Serial transplantation experiments with DOX-inducible ICN3I- expressing TE11 (TE11- ICN3 TetOn ). Tumor formation rates were determined as in Fig. 2e . * P < 0.05 vs. CD44L and DOX (−); n = 10. b Representative flow cytometry scatter plots of EPC2T cells with NOTCH3 -targeted or non-silencing (NS) control shRNA. NOTCH3 shRNA increased CD44H cells (lower right quadrant) to 29.8 ± 0.4% s.d. as compared to 0.4 ± 0.1% s.d. in NS control ( P < 0.0001 by Student’s t -test, n = 3). c qRT-PCR analysis for indicated genes comparing EPC2T cells with or without NOTCH3 knockdown. mRNA level for each gene in NS control cells was set to 1. * P < 0.05 vs. NS, n = 3. d Schematic of NOTCH3 second intron ( N3Int2 ) region and ChIP PCR primers in f and Supplementary Fig. 4e . Primers amplify the region lacking ZEB1 or CSL-binding sites. e Transfection assays for pGL3-N3Int2-luc reporter activity with or without ectopic ZEB1 or ZEB2 expression. bla , empty vector control for ZEBs. * P < 0.05 vs. bla and pGL3-luc (empty reporter); # P < 0.05 vs. bla and pGL3-N3Int2-luc ; ns not significant vs. bla and pGL3-N3Int2-luc ; n = 4. f ChIP assays for ZEB1 binding to N3Int2 region in purified CD44L and CD44H cells. CD44L cells were stimulated with TGFβ for 14 days to induce CD44H cells. * P < 0.0005 vs. CD44L and IgG and TGFβ (−); # P < 0.005 vs. CD44H and IgG and TGFβ (−); ** P < 0.05 vs. CD44L and anti-ZEB1 and TGFβ (+); ns not significant vs. IgG and TGFβ (−); n = 3. g Representative flow cytometry scatter plots of EPC2T cells with ZEB 1-targeted or NS control shRNA. * P < 0.05 vs. NS and TGFβ (−); # P < 0.0001 NS and TGFβ (+); ns not significant vs. NS and TGFβ (−); n = 3. In b , g , flow cytometry was done 7 days following lentivirus infection. All bar diagrams represent mean ± s.d. At least three independent replicates were performed for all experiments. Fisher’s exact test was used for percentage comparisons in a . Student’s t -test was used for paired data comparisons in b , c , f . ANOVA with Tukey’s post hoc test was used for multiple comparisons in e , g Full size image Notch1 at SCC invasive fronts predicts poor patient prognosis To demonstrate further the importance of Notch1 activity in pathogenesis of human SCCs, we analyzed surgically procured tissue samples (Supplementary Data 1 ) by immunohistochemistry (IHC) with two independent NOTCH1 antibodies, both detecting nuclear NOTCH1 at a 95.24% concordance rate ( κ = 0.664, 95% CI: 0.008–1.0, Kappa statistic, n = 21, Supplementary Fig. 5 ). ICN1 (ICN1 Val1744 ) was readily detectable in normal esophageal squamous epithelia ( n = 102) as described [4] and was upregulated in superficial precancerous as well as early invasive ESCC lesions (Supplementary Fig. 6 ). Within tumors invading into submucosa or muscularis propria, most SCC cells (>80%) did not express ICN1 with or without NOTCH1 mutations [6] , [7] ; however, a small subset of SCC cells expressed ICN1 in the invasive tumor front (35.3% for HNSCC, n = 17; 37.0% for ESCC, n = 227) (Fig. 7a ; Supplementary Fig. 6 ). Accompanied by desmoplastic stroma, ICN1-positive invasive SCC often displayed spindle-shaped cell morphology and ZEB1 co-localization (17.1%, n = 174) (Fig. 7a ; Supplementary Fig. 7 ) with ICN1 and ZEB1 expression being correlated ( ρ = 0.31, P < 0.0001, Pearson correlation). When stratified by co-localization status, expression of ICN1 and ZEB1 was relatively uncorrelated for subjects lacking co-localization ( ρ = −0.1, P = 0.2, Pearson correlation), while expression was correlated more strongly for those showing co-localization ( ρ = 0.37, P < 0.05, Pearson correlation, n = 30). Additionally, these cells were often found invading into lymphatic vessels (Fig. 7b ). NOTCH3 expression was low, if not absent, in SCC cells with concurrent ICN1 and ZEB1 expression (Supplementary Fig. 7 ). Moreover, ICN1 was expressed in a subset of ESCC cells with elevated CD44 expression (Fig. 7c ). 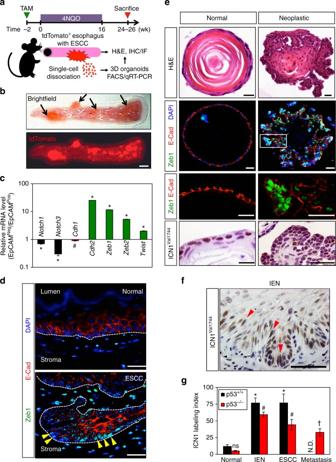Fig. 1 Lineage tracing reveals mesenchymal traits and Notch1 activation in ESCC lesions.aSchematic of cell-lineage tracing experiments.bMacroscopic and fluorescent images of representative tdTomato-labeled esophagus bearing 4NQO-induced tumors (arrows). Scale bar, 1 mm.cqRT-PCR analysis for indicated genes comparing EpCAMnegto EpCAMposcells from a representative tdTomato-labeled tumor. *P< 0.0001 and#P< 0.05 vs. EpCAMpos,n= 3.dRepresentative IF images for Zeb1 and E-cadherin (E-cad) in normal mucosa (top) and ESCC (bottom). Dashed line denotes interface between stroma and basal keratinocytes (top) or invasive ESCC cells (bottom). Note E-cadherin downregulation in ESCC cells with nuclear Zeb1 (arrowheads) at the tumor invasive front. Scale bar, 50 µm.eH&E, multicolor IF for E-cadherin and Zeb1, and IHC for ICN1 (ICN1Val1744) in representative single-cell-derived organoids from normal mucosa or 4NQO-induced tumors. Note that spherical organoids from 4NQO-untreated control mice exhibit a differentiation gradient with predominant luminal keratinization, whereas tumor-derived organoids (neoplastic) display irregular morphology with increased cellularity and diminished keratinization. Zeb1 expression was robust in tumor organoids, particularly at invasive protrusions with decreased E-cadherin expression and detectable ICN1 expression. Box denotes area magnified in panel below. Scale bars, 20 µm.fRepresentative IHC image for ICN1 4NQO-induced IEN (dysplasia) containing spindle-shaped cells (arrowheads). Scale bar, 50 µm.gQuantification of ICN1 IHC scoring in normal mucosa and 4NQO-induced lesions in mice of indicated genotype. *P< 0.05 vs.p53+/+(K5CreERT2;R26tdTomatolsl/lsl) normal,#P< 0.0005 vs.p53−/−(K5CreERT2;R26tdTomatolsl/lsl;p53loxP/loxP) normal;†P< 0.05 vs.p53−/−IEN; ns not significant vs.p53+/+normal. Data inb–frepresent at least three independent 4NQO-induced lesions and >20 organoids from at least two independent experimental replicates. Ing,n= 5 normal,n= 8 IEN, andn= 5 invasive ESCC in p53+/+esophagi. N.D. not detectable.n= 3 normal,n= 7 IEN,n= 5 invasive ESCC, andn= 4 metastatic tumors in p53−/−esophagi. Two independent experimental replicates were carried out. Bar diagrams represent mean ± s.d. incand mean ± s.e.m. ing. Student’st-test was used for paired data comparisons inc,g. ANOVA with Tukey’s post hoc test was used for multiple comparisons ing Evaluation of ICN1 in relation to clinicopathological data revealed that ICN1 was significantly associated with increased lymph node and distant metastases and advanced disease stages (Supplementary Table 1 ). Finally, analyses of clinical databases revealed that ICN1 expression at the invasive tumor front predicts independently for poor prognosis (Fig. 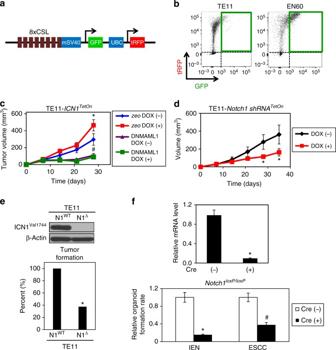Fig. 2 Notch1 promotes ESCC tumorigenesis.aSchematic of8×CSL-GFPreporter. Notch activation permits GFP reporter expression via concatemeric CSL-binding sites. Constitutively active UBC promoter drives tRFP expression concurrently. Cells without tRFP represent host-derived stromal cells.bRepresentative flow cytometry scatter plots determining8×CSL-mediated GFP reporter activation, indicating Notch active population of tRFP-labeled ESCC cells in TE11 and EN60 xenograft tumors. On average, 43.5 ± 0.5% s.d. of EN60 and 11.2 ± 6.5% s.d. of TE11 cells comprised the live GFPPos/tRFPPosfraction across three independent tumors.c,dTumor growth curves in immunodeficient mice carrying TE11 tumors of indicated genotypes. Upon xenograft transplantation, mice were treated with DOX to induceICN1orNOTCH1-directed shRNA. Tumor growth was monitored for indicated time periods. Inc, *P< 0.01 vs.zeoand DOX (−),#P< 0.05 vs.zeoand DOX (+),n= 6–8 per group. Ind, *P< 0.05 vs. DOX (−);n= 6 per group.eTE11 cells with CRISPR/Cas9-mediatedNOTCH1deletion. Immunoblotting confirms ICN1 loss inNOTCH1-deleted TE11 (N1Δ), but not non-targeted control TE11 (N1WT) cells. Bar graph shows tumor formation rate in immunodeficient mice 7 weeks after xenograft transplantation. *P< 0.05 vs. N1WT,n= 8 per group.fEsophageal keratinocytes isolated from 4NQO-induced IEN (dysplasia) lesions or ESCC tumors ofNotch1loxP/loxPmice were utilized to generate 3D esophageal organoids in the presence or absence of ex vivo Cre-mediated recombination. qRT-PCR analysis confirms inhibition ofNotch1gene expression upon ex vivo Cre-mediated recombination in ESCC organoids. *P< 0.000 vs. Cre (−),n= 3. Organoid formation rate was evaluated at day 14 post-plating and is represented as relative to Cre (−) for IEN and ESCC. *P< 0.000 vs. Cre (−) IEN;#P< 0.001 vs. Cre (−) ESCC. Line graphs represent mean ± s.e.m. inc,d. Bar diagrams represent mean ± s.d. inf. At least two independent replicates were performed for all experiments. Repeated measures ANOVA with Tukey’s post hoc test were used for multiple comparisons inc,d. Chi square with Fisher’s exact test was used for percentage comparisons ine. Student’st-test was used for paired data comparisons inf 7d ; Supplementary Table 2 ). Fig. 7 NOTCH1 activation and ZEB1 expression in invasive ESCC predicts poor prognosis. a , b Representative IHC images for ICN1 and ZEB1 in ESCC cells in a deep invasive tumor nest and ESCC cells invading into lymphatic vessels. a ESCC #55; b ESCC #62 in Supplementary Data 1 . c Representative IF image for ICN1 and CD44 in invasive ESCC cells. Scale bars, 50 μm in a – c . d Survival curve for 185 post-surgical ESCC patients with or without ICN1 expression at the tumor invasive front. e Model of the role of Notch1 in EMT in ESCC. Notch1 activation promotes tumorigenicity and heterogeneity in SCC via EMT. Notch1 drives squamous-cell differentiation by inducing Notch3 in normal squamous epithelia as well as SCC cells. Notch3 limits EMT. In response to TGFβ from the tumor microenvironment (e.g., cancer-associated fibroblasts and inflammatory cells), however, transcriptional repression of Notch3 by ZEB1 permits Notch1-mediated induction of CD44H cells via EMT. Notch activation may result in the generation and maintenance of CD44H cells possessing mesenchymal properties and enhanced malignant potential. EMT allows neoplastic cells to cope with stress during carcinogenesis and disease progression (e.g., genotoxic stress induced by 4NQO). CD44H cells produce pro-tumorigenic cytokines (e.g., IL-6) and tissue remodeling factors (e.g., MMP13, LOX, and POSTN) (Supplementary Fig. 3e ) Full size image The current study highlights an oncogenic role for Notch1 in SCC via EMT-mediated induction of CD44H cells with enhanced malignant potential (Fig. 7e ). We demonstrate that Notch1 and Notch3 may have opposing functions to allow expansion of CD44H cells both in vitro and in vivo. Moreover, we find that TGFβ guides Notch1 to drive EMT via a previously undescribed robust shift in the spectrum of Notch1 target genes including Notch3 , which is essential in squamous-cell differentiation [4] and senescence [12] , [48] . Given the microRNA-mediated crosstalk between Notch signaling and ZEB1 [33] , [49] , our findings indicate that direct repression of NOTCH3 by ZEB1 is a novel mechanism through which ZEB1 may influence Notch1-mediated cell fate determination. Activated Notch1 (i.e., ICN1) interacts with TGFβ downstream effector SMAD3 [45] . ZEB1 also binds physically to SMAD3 to enhance TGFβ-mediated transcription [34] . Additionally, ZEB1 promotes tumorigenicity by repressing stemness-inhibiting microRNAs in pancreas cancer [50] , where ZEB1 induction and EMT have been implicated as the earliest event preceding tumor formation in cell-lineage tracing experiments [51] . Taken together, these preclinical studies suggest that Notch1 and ZEB1 may cooperate to promote carcinogenesis and SCC progression via TGFβ-mediated EMT and offer the TGFβ–ZEB1–Notch1 axis as potential therapeutic target in SCC. Despite a well-established role for the Notch pathway in regulation of varied cell fates in a tissue-dependent and context-dependent manner, the molecular mechanisms governing Notch-mediated cell fate determination have yet to be fully elucidated. In non-transformed esophageal epithelium, Notch1-dependent transcriptional upregulation of Notch3 mediates squamous-cell differentiation as shown by us [4] . In the current study, we find Notch1 facilitates EMT-mediated expansion of CD44H cells with enhanced malignant potential. This raises the question of how Notch1 may act as a signal to induce both differentiation and dedifferentiation (i.e., EMT) in squamous epithelium. One potential explanation for this dichotomy is the influence of tissue microenvironment upon Notch-mediated cell fate determination. Indeed, microarray gene expression analysis in ICN1-overexpressing transformed esophageal keratinocytes indicates that TGFβ induces a dramatic shift in the spectrum of Notch1 target genes from a profile enriched for genes involved in squamous-cell differentiation to one consistent with EMT. Notch1 may also facilitate senescence in response to TGFβ in esophageal keratinocytes with intact cell cycle checkpoint functions [12] . The complexity in the role of Notch signaling in tumor biology is echoed by that of TGFβ as intratumoral cancer cell heterogeneity represents cancer cells that can respond to TGFβ and those cannot, the latter emerging during disease progression [52] . Thus, like TGFβ, Notch1 may have differential roles in cancer initiation and development. Besides TGFβ, hypoxia and inflammation may activate Notch1 to promote EMT in the tumor microenvironment via transcriptional factors such as HIF1α [17] and NF-κB [53] , respectively. Potential influence of these factors upon Notch1-mediated cell fates warrants further investigation in SCC as well as squamous epithelia under eosinophilic esophagitis where EMT and Notch3 downregulation are implicated (P.M.C. and H.N., unpublished observation). While our own published findings and those of others have implicated Notch1 as a tumor promoter in SCCs [12] , [54] , [55] , [56] , the current study is the first to demonstrate in vivo that Notch1 facilitates tumor initiation by converting CD44L cells to highly tumorigenic CD44H cells with mesenchymal traits, complementing the earlier studies implicating EMT and ZEB1 in the CD44L-to-CD44H transition [24] , [28] , [57] . While Notch1 activation and EMT were detected at the invasive tumor front, SCC cells with epithelial characteristics were commonly present in xenograft tumors, 4NQO-induced tumors, and human SCC samples. In our cell-lineage tracing experiments utilizing K5Cre ERT2 ;R26tdTomato lsl/lsl mice carrying 4NQO-induced tumors, complete loss of epithelial characteristics was uncommon, albeit present (Supplementary Fig. 1d ). Despite enhanced expression of mesenchymal-associated genes in EpCAM neg cells (Fig. 1c, d ), most tumors displayed a broad range of continuous EpCAM expression (Supplementary Fig. 1c ), suggesting a highly heterogeneous and plastic nature of SCC cells. Besides squamous-cell differentiation, Notch3 may be permissive for mesenchymal–epithelial transition or epithelial–mesenchymal hybrid characteristics of cancer cells by limiting EMT [58] , [59] . These findings have potential clinical impact as reducing CD44H cells may delay disease progression or post-therapeutic recurrence and increase sensitivity to chemotherapeutic agents, providing a platform for new human clinical trials. Given the interplay between Notch1 and Notch3 in regulating esophageal cell fate, the use of pan-Notch inhibitors may prove problematic. Indeed, genetic Notch inhibition via DNMAML1 expression accelerates carcinogen-mediated esophageal tumor initiation, growth and invasion in vivo [60] , [61] . Tumor initiation by CD44H cells may be independent of Notch because purified CD44H cells gave rise to tumors with or without DOX-induced ICN1 expression or in the presence of DNMAML1 (Fig. 3c ). Interestingly, Notch inhibition by DNMAML1 permits clonal immortalization and expansion of murine esophageal epithelial cells [61] . Thus, Notch1 activation is essential for the induction of CD44H cells while it may be dispensable for their maintenance and tumor initiation by CD44H cells. Such a premise is corroborated by ICN1 expression localized to tumor invasive fronts, but not in the majority of expanding ESCC cell populations (Supplementary Fig. 6 ). Notch signaling can be selectively modulated by Notch receptor paralog-specific antibodies [62] , [63] . TGFβ signaling can be also regulated by TGFβ inhibitors [64] . Notably, the observed inhibitory effects of anti-TGFβ antibody upon tumor progression in mice (Fig. 4 ) may involve TGFβ downstream effectors other than Notch1, representing a limitation of the current study. Since TGFβ-induced EMT involves autophagy in ESCC cells where pharmacological inhibition of autophagy flux by chloroquine decreases CD44H cells, an alternative approach to target EMT and CD44H cells [30] . Future studies evaluating the efficacy of these agents in SCC therapy are currently underway in preclinical models. Technical innovation in this study includes use of a HNSCC PDX model as well as a cell-lineage tractable mouse model of ESCC through which EMT was for the first time documented unequivocally in SCC cells in situ. Additionally, we have developed an esophageal 3D organoid platform that recapitulates esophageal tissue architecture ex vivo and can be utilized to model esophagitis [65] . Here, we apply this model system to SCC, generating murine ESCC-derived 3D organoids for the first time (Fig. 1e ). Upon ex vivo culture, single-cell-derived 3D organoids from 4NQO-induced dysplasia and ESCC tumors display morphological characteristics of neoplastic epithelium, including nuclear atypia, perturbed squamous-cell differentiation and evidence of EMT, which are maintained upon organoid passaging (K.A.W., P.M.C., and H.N., unpublished observation). We have also successfully performed ex vivo Cre-mediated recombination in 3D organoids generated from neoplastic esophageal keratinocytes of 4NQO-treated Notch1 loxP/loxP mice, demonstrating that Notch1 is required for organoid formation and EMT-like features in neoplastic 3D organoids (Figs. 2 f, 3e ). Notch1 deletion in the murine skin promotes SCC development in a non-cell autonomous fashion due to inflammation associated with epidermal barrier defects [5] , limiting the assessment of the cell-autonomous oncogenic role of Notch1 in vivo. The 3D organoid system provides insights about cell-autonomous oncogenic functions of Notch1 in the absence of inflammatory milieu ex vivo, complementing in vivo experiments. The 4NQO model requires a long-term 4NQO administration (16 weeks) where tumors arise 6–9 weeks after 4NQO withdrawal during the observation period; however, it is not precisely known when malignant transformation occurs in this model. The single-cell-derived 3D organoids have a potential to detect neoplastic changes in a more sensitive and quantitative manner than conventional morphological tissue assessment. Such a study is underway. Once an appropriate window of 4NQO-induced malignant transformation is determined, our cell-lineage traceable mice can be utilized for genetic ablation of Notch1 following 4NQO administration to elucidate how Notch1 may exert its oncogenic role by promoting EMT and tumor initiation and/or progression in vivo. Alternatively, such mice may be treated with Notch1-specific antagonistic antibody [63] or anti-Notch3 agonistic antibody [62] , the latter can be used for targeted activation of Notch3. While these findings identify 3D neoplastic organoids as sustainable resource for functional and mechanistic investigations into the biology of ESCC, it remains to be determined how faithfully organoid genetics and biology mimic that of the tissue from which they are derived upon extended ex vivo culture. Ongoing studies include procuring of a bank of human patient-derived ESCC 3D organoids that may be utilized as an experimental platform for discovery and validation of novel translational applications for prognosis and therapy in the setting of personalized medicine. Taken together, the current study supports a tumor-promoting role of Notch1 in SCC while also providing novel mechanistic insight into how the local tissue microenvironment may influence Notch-mediated cell fate determination. Patients and tissue samples Surgically removed tissue samples (Supplementary Data 1 ) were described previously [11] , [66] , [67] , [68] or newly procured at Kagoshima University Hospital in accordance with Institutional Review Board standards and guidelines. Informed consent was obtained from all human subjects. Most samples were available as tissue microarrays (TMAs) [67] , [68] containing primary ESCC ( n = 171), carcinoma in situ (CIS; n = 9), IEN ( n = 7), and normal mucosa ( n = 114). Samples with NOTCH1 mutations ( n = 4; E755*, D469Y, R1279D, and D1457G) and wild-type NOTCH1 ( n = 15) were identified by DNA sequencing (SRP072948) [69] . Given the limitation of TMAs to assess intratumoral cancer cell heterogeneity [70] , we examined whole paraffin blocks ( n = 244) by Hematoxylin and Eosin (H&E) staining and IHC, as described below, following preliminary analysis with TMAs. Survival analysis was done on IHC data for 185 ESCC patients who did not receive chemotherapy or radiation therapy prior to surgery. Esophageal epithelial cell-lineage traceable mice and 4NQO treatment The K5Cre ERT2 transgenic mouse strain [68] was intercrossed with R26tdTomato lsl/lsl (Jackson Laboratory, Bar Harbor, ME) carrying the homozygous Rosa26 locus with knocked-in tdTomato fluorescent protein as a reporter under the loxP-stop-loxP sequence. The resulting K5Cre ERT2 ;R26tdTomato lsl/wt mice were crossed with R26tdTomato lsl/lsl mice to generate K5Cre ERT2 ; R26tdTomato lsl/lsl mice. Similarly, K5Cre ERT2 ;p53 loxP/loxP mice were generated with p53 loxP/loxP mice (Jackson Laboratory). R26tdTomato lsl/lsl mice were also crossed with p53 loxP/loxP to generate R26tdTomato lsl/wt ;p53 loxP/wt mice, which were then crossed to generate R26tdTomato lsl/lsl ;p53 loxP/loxP mice. The K5Cre ERT2 ;p53 loxP/loxP mice were further crossed with R26tdTomato lsl/lsl ;p53 loxP/loxP mice to generate K5Cre ERT2 ;R26tdTomato lsl/wt ;p53 loxP/loxP . These mice were further crossed with R26tdTomato lsl/lsl ;p53 loxP/loxP to generate and maintain the K5Cre ERT2 ;R26tdTomato lsl/lsl ;p53 loxP/loxP strain. The L2Cre transgenic mouse strain [71] was intercrossed with p53 R172H/R172H mice [72] to generate L2Cre;p53 R172H/wt mice. We administered TAM (Sigma-Aldrich, St. Louis, MO; 0.25 mg/g body weight) via oral gavage to 3–4-month-old K5Cre ERT2 ;R26tdTomato lsl/lsl and K5Cre ERT2 ;R26tdTomato lsl/lsl ; p53 loxP/loxP littermates 2 weeks before starting 4-Nitroquinoline N -oxide (4NQO) (Sigma-Aldrich) treatment. Mice received 100 µg/ml 4NQO in 2% propylene glycol (MP Biomedicals, Solon, OH) in drinking water for 16 weeks and were followed up for 8–10 weeks (or earlier if mice were ill) after 4NQO withdrawal as described [73] . To inhibit TGFβ receptor-mediated signaling, mice were treated for 2 weeks with either anti-TGFβ antibody 1D11 (intra-peritoneally), neutralizing all three isoforms of TGFβ [46] (a gift of Dr. Singhal, University of Pennsylvania; 3 mg/kg, three times per week) or control IgG (intra-peritoneally) with injections initiated 4 weeks following 4NQO withdrawal. At the time of sacrifice, one half of the dissected esophagus or a tumor (if visible macroscopically) from each mouse was fixed in 4% paraformaldehyde and paraffin-embedded for morphological analyses. The other half of esophagi and tumors was dissociated as described previously [74] and cell suspensions were subjected to flow cytometry or FACS and organoid formation assays. All experiments were done under approved protocols from the University of Pennsylvania Institutional Animal Care and Use Committee (IACUC). Sample size for groups were projected based on data from pilot studies. Animals were only excluded from analyses in event of death from procedure-related causes (e.g., death following oral gavage) that were unrelated to experimental differences between groups. Animals were randomized to treatment groups with consideration given to representation of both sexes. Investigators were informed of groups during treatment phase of experiments. Upon processing, tissues were given a unique identifier to blind investigators during analyses and outcome assessments. Xenograft transplantation experiments Xenograft transplantation experiments were done as described [11] , [12] . In brief, 1–5 × 10 6 cells were suspended in 50% Matrigel and implanted subcutaneously into the dorsal skin of female athymic nu / nu mice (4–6 weeks old; Charles River Breeding Laboratories). PDX tumor transplantation was performed as previously described with fragments of passaged PDX tumors implanted under the dorsal skin of NOD/SCID/IL2 receptor γ-chain-deficient (NSG) mice [75] . Tumor growth was monitored and mice were sacrificed 6–10 weeks after inoculation for flow cytometry and histopathological analyses. One half of each tumor was fixed in formalin and embedded in paraffin blocks. The other half of each tumor was enzymatically dissociated and subjected to flow cytometry and FACS for serial transplantation experiments where 10–10 3 cells were injected into recipient mice to determine tumor formation rates. For tetracycline/DOX-inducible (TetOn) transgene expression in xenograft tumors, mice were fed daily with DOX-containing pellets (20 mg/kg). To inhibit TGFβ receptor-mediated signaling, mice were treated for 2 weeks with either anti-TGFβ antibody 1D11 (intra-peritoneally) (3 mg/kg, 2–3 times per week) or control IgG (intra-peritoneally), beginning when tumor volume reached 60 mm 3 . All experiments were approved by the University of Pennsylvania IACUC or under Wistar Institute IACUC protocols 112652/112655. Sample size for groups were projected based on previous xenograft studies then adjusted following acquisition of data in initial experiment. Animals were only excluded from analyses in event of death from procedure-related causes (e.g., sepsis) that were unrelated to experimental differences between groups. Animals were randomized by cage upon arrival. Investigators were informed of groups during treatment phase of experiments. Upon processing, tumors were given a unique identifier to blind investigators during analyses and outcome assessments. DNA constructs A lentiviral vector pTRIPZ expressing DOX-inducible shRNA directed against human NOTCH1 (Notch1-A; V2LHS_149557 and Notch1-B; V3LHS_637133) and pTRIPZ-NS carrying a non-silencing scrambled sequence (RHS4346) (GE Dharmacon, Lafayette, CO) were purchased. Other shRNA sequences in pGIPZ (GE Dharmacon) targeting NOTCH3 (Notch3-A; V2LHS_229748 and Notch3-B; V2LHS_93017), ZEB1 (ZEB1-A; V2LHS_116663 and ZEB1-B; V2LHS_116659), and a non-silencing scrambled sequence (RHS4348) were used as described previously [11] , [12] , [19] . To generate a lentiviral vector pTR-tRFP expressing constitutively turbo RFP ( tRFP ) under ubiquitin C (UBC) promoter, a DOX-inducible gene expression vector pTRIPZ-MCS [12] was modified by removal of Bam HI and LoxP sites and a subsequent insertion of new multiple cloning sites (MCS) comprising 5′- Age I- Bam HI- Sna BI- Eco RI- Xho I- Mlu I-3′, resulting in the creation of pTRIPZ-MCS2. We then amplified an open reading frame (ORF) for turbo RFP ( tRFP ) by PCR using pTRIPZ-NS (RHS4743, GE Dharmacon) as a template with primers 5′-AGCGCTAGCGCCACCATGAGCGAGCTGATC-3′ and 5′-AGCGCGGCCGCTTATCTGTGCCCCAGTTTGCTAGG-3′. Following removal of rtTA-encoding ORF flanked by Nhe I and Not I sites, the purified tRFP ORF was subcloned into the Nhe I and Not I sites of pTRIPZ-MCS2, resulting in creation of pTR-tRFP. To generate a lentiviral vector carrying 8×CSL-GFP reporter, an ORF for GFP was isolated from pBABE-zeo-GFP [19] and ligated into the EcoR I and Xho I sites of pTR-tRFP, generating pTR-tRFP-GFP. A DNA fragment containing a concatemer of eight copies of CSL-binding sites fused to minimal SV40 (mSV40) promoter was isolated from 8× CSL-luc [76] by PCR with primers 5′-AGCTCTAGACTCTTACGCGT GCTAGCTCGA-3′ and 5′-AGCACCGGTTTTGCAAAAGCCTAG GCCTCCA-3′ to replace the sequence containing tetracycline response elements and minimal CMV promoter from pTR-RFP-GFP at the Xba I and Age I sites, resulting in a creation of pTR-RFP-8×CSL-GFP. To delete human NOTCH1 via Crispr/Cas9-mediated gene editing, five candidate guide RNA (gRNA) sequences were subcloned into lentiCRISPR v1 (gift of a gift from Feng Zhang; Addgene, plasmid #52961) at its Bsm BI sites and used as described [77] . gRNAs 1, 2, and 5 targeting chromosome 9 NOTCH1 exon 14 (EGF-like region at 139,407,894–139,407,913) or exon 19 (EGF-like region at 139,403,465–139,403,484) and exon 34 (PEST domain at 139,390,539–139,390,558), respectively, were found to be equally effective to delete NOTCH1 . To generate a retroviral vector BABE-zeo-FLAG-DNMAML1, we amplified an Flag-MAML1 1–302 ORF by PCR using pFLAG-CMV2-MAML1 (1–302) (a gift from Dr. Wu, University of Florida) as a template with primers 5′-GCACGGATCCGCCACCATGGACTACAAAGACGATGA CGACAAG-3′ and 5′-GCACGTCGACCTAGAATTCCGTCTTAATATTAATGTCCTGTGCC-3′ and subcloned at the Bam HI and Sal I sites of pBABE-zeo [78] . To generate pBABE-bla-ZEB1 and pBABE-bla-ZEB2, ZEB1 and ZEB2 ORFs in pCR-BluntII-TOPO were purchased from GE Dharmacon (clone 40036600 for ZEB1 and clone 40124124 for ZEB2). The ZEB1 and ZEB2 ORFs were amplified by PCR with primers 5′-CGCTGGATCCGCCGCCACCATGGCGGATGG CCCCAGGTG-3′ and 5′-CGGAGTCGACTTAGGCTTCATTTGTCTTTTC-3′ for ZEB1 and 5′-CG CTGGATCCGCCGCCACCATGAAGCAGCCGATCATGGC-3′ and 5′-CGGAGTCGACTTACATGCCATCTTCCATATTG-3′ for ZEB2, respectively, and subcloned at the Bam HI and Sal I sites of pBABE-bla [79] . The 2nd intron of NOTCH3 ( N3Int2 ) containing ZEB1-binding sites (488-bp) was amplified by PCR using the input DNA sample from ChIP assay as a template with primers 5′-GGGAGATCTGGTTCCCACGCTCTGCGTCC-3′ and 5′-GGGCTCGAGCCGCGCCTGGAATACTGCCG-3′. Then the amplified DNA was subcloned at the Xho I and Bgl II sites of pGL3 promoter (Promega, Madison, WI), creating a plasmid pGL3-N3Int2-luc. All constructs were verified by DNA sequencing. Cell culture, genetic modifications, and pharmacological treatments of cells TE11, EN60, EPC2T, and derivatives were grown at 37 °C in a 5% CO 2 atmosphere as described previously [12] . Additional genetic modifications were done via stable gene transfer of the above retroviral and lentiviral constructs as described previously [12] . Stable cell lines were established by drug selection for 7 days with 1 µg/ml of Puromycin (Invitrogen) for genes transduced via pTRIPZ or lentiCRISPR; and 0.5 µg/ml zeocin (Invitrogen) for Flag-MAML1 1–302 transduced via pBABE-zeo. Cells transduced with GFP (pGIPZ) or tRFP (pTR-tRFP) were selected for the brightest level of fluorescence (top 20%) by FACS. EPC2T, EN60, and derivatives were kept undifferentiated in Keratinocyte serum-free medium (Invitrogen, Carlsbad, CA) containing a low concentration (0.09 mM) of CaCl 2 . Squamous-cell differentiation was induced by 0.6 mM CaCl 2 (Sigma-Aldrich) as described [4] . Compound E (Calbiochem, La Jolla, CA), a GSI, and SB431542 (Calbiochem), a TGFβ type I receptor kinase inhibitor were reconstituted in dimethyl sulfoxide (DMSO) (Sigma-Aldrich). Cells were treated with 1 µM Compound E or 5 ng/ml recombinant human TGFβ1 (R&D Systems, Minneapolis, MN) as optimized previously [4] , [19] , [80] . SB431542 was used at 10 µM. Dox was used at 1 µg/ml for DOX-inducible transgene expression [12] . Phase contrast images were acquired using a Nikon Eclipse E600 microscope. EPC2-hTERT cells and derivatives were established and extensively characterized by us [12] , [30] , [74] . TE11 [12] , [30] , [81] and EN60 [12] , [82] cells were generous gifts from Dr. Tetsuro Nishihira (Tohuko University, Sendai, Japan) and Dr Hiroshi Shirasawa (Chiba University, Chiba, Japan), respectively, and were extensively characterized by us [12] , [30] , [74] , [83] . The earliest frozen stocks of all cell lines have been stored at the Cell Culture Core of the University of Pennsylvania. We have propagated cells from frozen stocks of original vials that were authenticated by short tandem repeat profiling (ATCC) for highly polymorphic microsatellites to validate the identity of cells by comparing cells at the earliest stocks and those grown >8–12 passages. All cell lines undergo routine mycoplasma testing. Organotypic 3D culture OTC was carried out as described previously [74] . In brief, 0.5 × 10 6 of epithelial cells were seeded on top of the collagen/Matrigel matrices containing FEF3 human fetal esophageal fibroblasts, and grown in submerged conditions for 4 days. Cultures were then raised to the air–liquid interface for additional 4 days and harvested for morphological assessment. Each OTC experiment was performed in triplicate. Ex vivo esophageal organoid 3D culture Esophageal keratinocytes were isolated from vehicle-treated or 4NQO-treated K5Cre ERT2 ;R26tdTomato lsl/lsl or Notch1 loxP/loxP (Jacskon Laboratories) mice under an IACUC-approved protocol as described previously [65] , [84] , [85] . Using 24-well plates, 5000 cells were seeded per well in 50 μl Matrigel. After solidification, 500 μl of DMEM/F12 supplemented with 1× Glutamax, 1× HEPES, 1× N2 Supplement, 1× B27 Supplement, 0.1 mM N -acetyl-L-cysteine (Sigma-Aldrich), 50 ng/ml mouse recombinant EGF (R&D Systems), 2.0% Noggin/R-Spondin-conditioned media and 10 μM Y27632 (Tocris Biosciences, Bristol, UK) were added and replenished every other day. For ex vivo recombination, organoids were cultured in the presence of Adenovirus vector containing Cre recombinase and GFP (University of Iowa Gene Transfer Vector Core). Adenovirus vector containing GFP alone was used as a control. Adenovirus vectors were used at 1:500 at the time of organoid plating. Organoid formation rate was calculated as the percentage of the number of organoids formed at day 7 per total number of cells seeded at day 0. After 14 days organoids were recovered by digesting Matrigel with Dispase I (BD Biosciences, San Jose, CA; 1 U/ml) and fixed overnight in 4.0% paraformaldehyde. Specimens were embedded in 2.0% Bacto-Agar: 2.5% gelatin prior to paraffin embedding. RNA isolation, cDNA synthesis, qRT-PCR, and microarray analyses RNA isolation, cDNA synthesis, and qRT-PCR were done using StepOnePlus™ Real-Time PCR System (Applied Biosystems) by TaqMan ® Gene Expression Assays (Applied Biosystems) for NOTCH1 (Hs01062014_m1), Notch1 (Mm00435249_m1), NOTCH3 (Hs00166432_m1), Notch3 (Mm00435270_m1), IVL (Hs00846307_s1), CK13 (s00999762_m1), CDH1 (Hs00170423_m1), CDH2 (Hs00983062 _m1), ZEB1 (Hs00232783_m1), SNAI1 (Hs00195591_m1), and PAI1 (Hs01126606_m1), and SYBR ® Green PCR for human ACTB (β-Actin) as well as murine Cdh1 (5′-TCAAGCTCGCGGATAACCAGAACA-3′ and 5′-ATTCCCGCCTTCATGCAGTTGTTG-3′), Cdh2 (5′-ATGGCCTTTCAAACACAGCCACAG-3′ and 5′-ACAATGACGTCCACCCTGTTCTCA-3′), Zeb1 (5′-TGAGCACACAGGTAAGAGGCC-3′ and 5′-GGCTTTTCCCCAGAGTGCA-3′), Zeb2 (5′-TGATAGCCTTGCAAACCCTCTGGA-3′ and 5′-TCCTTCATTTCTTCTGGACCGGCT-3′), Twist (5′-AGCTGAGCAAGATTCAGACCCTCA-3′ and 5′-TGCAGCTTGCCATCTTGGAGT-3′), and Gapdh (5′-GGTGGTCTCCTCTGACTTCAACA-3′ and 5′-GTTGCTGTAGCCAAATTCGTTGT-3′) and as described [4] , [11] , [19] . All PCR reactions were performed in triplicate. The relative level of each mRNA was normalized to ACTB (β-actin) for human genes and Gapdh for murine genes as internal controls. Gene array experiments were done using an Affymetrix gene chip (U133+v2.0) (Affymetrix, Santa Clara, CA) as described [11] , [31] . Data were deposited at the NCBI Gene Expression Omnibus ( http://www.ncbi.nlm.nih.gov/geo ) (accession #GSE37994). Immunoblot analysis Whole cell lysates were prepared as described [4] , [11] . 20 μg of denatured protein was fractionated on a NuPAGE Bis-Tris 4–12% gel (Invitrogen). Following electrotransfer, Immobilon-P membranes (Millipore) were incubated with primary antibodies for rat monoclonal anti-NOTCH1 5B5 (1:1000; 3447, Cell Signaling, Danvers, MA), rabbit monoclonal anti-ICN1 Val1744 D3B8 (1:1000; 4147, Cell Signaling), rat monoclonal anti-NOTCH3 8G5 (1:1000; 3446, Cell Signaling), mouse monoclonal anti-E-cadherin (1:10,000; 610182, BD Biosciences), mouse monoclonal anti-N-cadherin clone 32 (1:1000; 610920, BD Biosciences), mouse monoclonal anti-Involucrin clone SY5 (1:1000, I9018, Sigma-Aldrich) and mouse monoclonal anti-β-actin (1:10,000; AC-74, Sigma-Aldrich), and then with the appropriate HRP-conjugated secondary antibody (GE Healthcare, Piscataway, NJ). β-actin served as a loading control. Uncropped images of blots from primary figures are shown in Supplementary Fig. 8 . Flow cytometry and FACS Flow cytometry and FACS were performed as described previously [86] . FACSCalibur or LSRII (BD Biosciences, San Jose, CA) and FlowJo (Tree Star, Ashland, OR) were used for flow cytometry. FACS Vantage SE and FACS Aria II (BD Biosciences) were used to sort purified CD44 high -CD24 low/− cells (CD44H) and CD44 low/− -CD24 high cells (CD44L) from EPC2T, TE11 and EN60 cells, and/or xenograft tumors. Cells were suspended in Hank’s balanced salt solution (Invitrogen) containing 1% BSA (Sigma-Aldrich) and stained with the following antibodies on ice for 30 min: human PE/Cy7-anti-CD24 clone [ML5] (1:40; 311,120, BioLegend, San Diego, CA), human APC-anti-CD44 clone G44-26 (1:20; 559,942, BD Biosciences), human FITC-anti-CD326 (EpCAM) clone HEA-125 (1:50; 130-089-113, Miltenyi Biotec, San Diego, CA) and/or mouse APC-Cy7-anti-CD326 (EpCAM) Clone G8.8 (1:50; 118,217, BioLegend). 4′,6-diamidino-2-phenylindole (DAPI; 2 μg/μl; Invitrogen) was used to assess viability. CD44T cells were defined as CD44 high -CD24 High . To purify CD44L and CD44H cells from TE11 and EN60 xenograft tumors, tumors were minced into 1 mm 3 pieces and incubated in Dulbecco’s Modified Eagle Medium (DMEM; Invitrogen) containing 1 mg/ml collagenase I (Sigma-Aldrich) at 37 °C for 90 min. Following centrifugation, residual tissue pieces were digested in 0.05% trypsin-EDTA (Invitrogen) at 37 °C for 10 min and then with 1 U/ml Dispase (BD Biosciences) and 100 μg/ml DNase I (#10104159001, Roche) at 37 °C for 10 min. Dissociated tumor cells were filtered with a 40 µm cell strainer (BD Biosciences) and washed prior to incubation with antibodies. Cancer cells were distinguished from host-derived stromal cells by tRFP expression detected concurrently. In 8×CSL-GFP reporter assays, tRFP-positivity was used to identify human cells while GFP expression was monitored to evaluate Notch activity. In tissue from 4NQO-treated mice and controls, tdTomato expression was used to isolate epithelial cells that had undergone K5Cre ERT2 -mediated recombination following TAM treatment. Following dissection, esophagi were incubated with 1 U/ml Dispase for 5 min at 37 °C then epithelial layer was peeled from underlying stroma using fine tipped forceps. Epithelia were then incubated in 0.25% trypsin two times for 5 min at 37 °C with agitation to liberate keratinocytes. Trypsin was quenched with soybean trypsin inhibitor then liberated cells were filtered with a 40 µm cell strainer prior to staining. Flow cytometry was repeated for each genotype and condition at least three times. Immunofluorescence (IF) and IHC IF and IHC for NOTCH1, NOTCH3, ZEB1, E-cadherin, CD44, and tdTomato were done as described previously [4] , [11] , [12] . IHC for Notch1 was done with two independent anti-NOTCH1 antibodies, namely, polyclonal rabbit polyclonal anti-NOTCH1 (ab27526; Abcam; 1:250) and rabbit polyclonal anti-ICN1 V1744 (2421; Cell Signaling; 1:100), both detecting cytoplasmic and nuclear expression of NOTCH1. The following primary antibodies were used for IHC and/or IF: rabbit polyclonal anti-NOTCH3 (ab23426; Abcam; 1:250), rabbit polyclonal anti-ZEB1 (a generous gift from Dr. Darling, University of Louisville; 1:100), mouse monoclonal anti-E-cadherin (610182; BD Biosciences; 1:100), rabbit polyclonal anti-RFP (ab34771, Abcam; 1:100). IHC signals were developed using the diaminobenzidine substrate kit (Vector Laboratories, Burlingame, CA) following incubation with secondary anti-mouse IgG (Vector; 1:600 at 37 °C for 30 min) or anti-rabbit IgG (Vector; 1:600 at 37 °C for 30 min), and counterstained with Hematoxylin (Fisher Scientific CS401-1D). 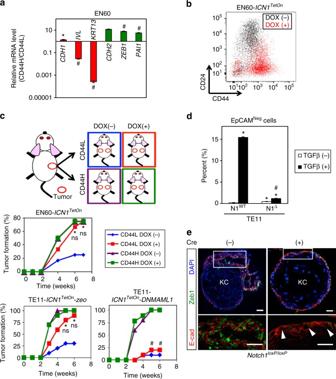Fig. 3 Notch1 facilitates expansion of CD44H cells with mesenchymal properties.aqRT-PCR analysis for indicated genes comparing EN60 intratumoral CD44L and CD44H cells. *P< 0.05 vs. CD44L;#P< 0.0001 vs. CD44L;n= 3 per group.bRepresentative flow cytometry scatter plot determining CD44H cells in EN60 tumors grown for 4 weeks with or without DOX-induced ICN1 (EN60-ICN1TetOn).cExperimental design of serial transplantation experiments and tumor formation rates by CD44L and CD44H cells purified from parental xenograft tumors carrying DOX-inducibleICN1(EN60-ICN1TetOnand TE11-ICN1TetOn). Parental tumors were grown in mice without DOX treatment and dissociated for FACS-purification of CD44L and CD44H cells. Purified cells were serially transplanted (103cells per injection site) into recipient mice to monitor tumor formation. Recipient mice were treated with or without DOX. TE11 carriedDNMAML1orzeo(empty vector control). *P< 0.05 for CD44L and DOX (+) vs. CD44L and DOX (−),n= 10–12 per group; ns not significant for CD44L and DOX (+) vs. CD44H (with or without DOX treatment),n= 10 per group;#P< 0.05 vs. TE11-ICN1TetOn-zeoCD44L and DOX (+),n= 10 per group.dFlow cytometry analysis for EpCAM-negative cells in TE11 withNOTCH1deletion (N1Δ) or wild-type control (N1WT). Cells were treated with or without 5 ng/ml TGFβ for 72 h. *P< 0.05 vs. TGFβ (−);#P< 0.0001 vs. N1WTand TGFβ (+),n= 3. Data are presented as mean ± s.e.m.eMulticolor IF for E-cadherin and Zeb1 in representative single-cell-derived organoids from 4NQO-induced ESCC tumors ofNotch1loxP/loxPmice with or without ex vivo Cre-mediated recombination. Zeb1 expression diminished in organoids upon Cre-mediated Notch1 deletion (arrowheads). Box denotes area that is magnified in panel below. KC keratinized core of organoids. Scale bars, 20 µm. Bar diagrams represent mean ± s.d. ina,d. At least two independent replicates were performed for all experiments. Student’st-test was used for paired data comparisons ina,d. Chi square with Fisher’s exact test was used for percentage comparisons inc For IF, Cyanine Cy2-conjugated or Cyanine Cy3-conjugated affinity-purified anti-mouse or anti-rabbit IgG (Jackson Immuno-Research; 1:600) was used for signal detection by incubating at 37 °C for 30 min, and cell nuclei were counterstained by DAPI (Invitrogen; 1:10,000). 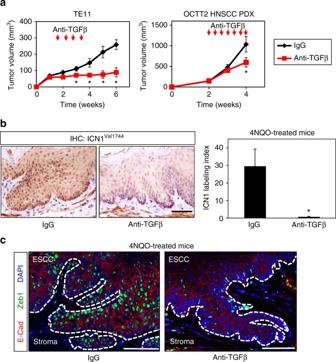Fig. 4 TGFβ signaling facilitates ESCC tumor growth, Notch1 signaling, and EMT.aGrowth curve for mice bearing TE11 or HNSCC PDX tumors receiving either ID11 anti-TGFβ blocking antibody or control IgG via intraperitoneal injection at indicated time points (arrows). ID11 neutralizes all TGFβ isoforms. *P< 0.05 vs. IgG,n= 5–8 per group.b,cp53+/+mice were treated with 4NQO for 16 weeks. Six weeks following 4NQO withdrawal, mice were treated with ID11 anti-TGFβ blocking antibody or control IgG via intraperitoneal injection three times weekly for a period of 2 weeks. Inb, quantification of ICN1 IHC scoring in esophageal epithelium with representative IHC images for IgG-treated and anti-TGFβ blocking antibody-treated animals. *P< 0.05;n= 4–5 per group. Scale bar, 50 µm. Inc, multicolor IF for E-cadherin and Zeb1 in representative 4NQO-induced IEN lesions from IgG-treated and anti-TGFβ blocking antibody-treated animals. Data indicate mean ± s.e.m. ina,b. At least two independent replicates were performed for all experiments. Repeated measures ANOVA with Tukey’s post hoc test were used for multiple comparisons ina. Student’st-test was used for paired data comparisons inb Stained objects were examined with a Nikon E600 microscope and imaged with a digital camera. The staining was assessed independently by pathologists (S.N. and A.K.S. 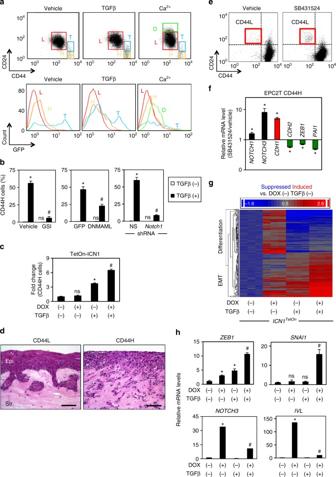Fig. 5 TGFβ-mediated Notch1 activation permits EMT and suppresses differentiation.aRepresentative flow cytometry scatter and histogram plots for8×CSL-GFPreporter activity in indicated subpopulations of EPC2T cells treated with TGFβ or CaCl2for 72 h.b,cFlow cytometry determined CD44H cells induced in FACS-purified CD44L cells with indicated conditions or genotypes. Cells were treated with TGFβ or DOX for 7 days. *P< 0.0001 vs. TGFβ (−);#P< 0.005 vs. TGFβ (+) and DMSO,GFP, or non-silencing scrambled (NS) shRNA inb;n= 3. *P< 0.05 vs. TGFβ (−) and DOX (−); ns not significant vs. TGFβ (−) and DOX (−);#P< 0.05 vs. TGFβ (+) and DOX (−) inc;n= 3.dRepresentative H&E images of OTC reconstituted with CD44L or CD44H cells. Epi epithelia, Str stroma. Scale bar, 50 μm.eRepresentative flow cytometry scatter plots of purified CD44H cells treated with SB431542 or vehicle (control) for 14 days. SB431542 increased CD44L cell content (upper left quadrant) to 0.35 ± 0.08% as compared to 1.2 ± 0.1% s.d. in vehicle (P< 0.0005,n= 3).fqRT-PCR analysis for indicated genes in FACS-purified CD44H cells treated with or without SB431542. mRNA level for each gene in vehicle-treated cells was set as 1. *P< 0.0005 vs. vehicle,n= 3.gHeat map of gene array results from EPC2T derivative (EPC2T-ICN1TetOn) treated with DOX and/or TGFβ (n= 3 per condition). “Differentiation” genes were significantly increased (≥1.5-fold) by DOX-induced ectopic ICN1 alone, but suppressed by TGFβ (P< 0.05 by two-way ANOVA). “EMT” genes activated by TGFβ (≥1.5-fold) were significantly augmented by ectopic ICN1 (P< 0.05 by two-way ANOVA).hqRT-PCR analysis validates gene array results ing. mRNA level for DOX (−) and TGFβ (−) was set to 1. *P< 0.001 vs. TGFβ (−) and DOX (−);#P< 0.0001 vs. TGFβ (−) and DOX (+); ns not significant vs. TGFβ (−) and DOX (−);n= 3. All bar diagrams indicate mean ± s.d. Student’st-test was used for paired data comparisons ine,f. At least two independent replicates were performed for all experiments. ANOVA with Tukey’s post hoc test were used for multiple comparisons inb,c,h ), and the intensity was expressed as negative (0), marginally positive (0.5), weakly positive (1), moderately positive (2), or strongly positive (3). Both antibodies detect cytoplasmic and nuclear NOTCH1 at high concordance rates, although anti-ICN1 V1744 antibody was more sensitive than ab27526 to detect nuclear Notch1 expression (Supplementary Fig. 5 ). 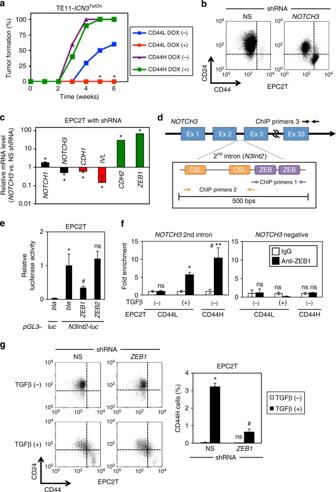Fig. 6 ZEB1 repressesNOTCH3, facilitating EMT and tumor initiation.aSerial transplantation experiments with DOX-inducibleICN3I-expressing TE11 (TE11-ICN3TetOn). Tumor formation rates were determined as in Fig.2e. *P< 0.05 vs. CD44L and DOX (−);n= 10.bRepresentative flow cytometry scatter plots of EPC2T cells withNOTCH3-targeted or non-silencing (NS) control shRNA.NOTCH3shRNA increased CD44H cells (lower right quadrant) to 29.8 ± 0.4% s.d. as compared to 0.4 ± 0.1% s.d. in NS control (P< 0.0001 by Student’st-test,n= 3).cqRT-PCR analysis for indicated genes comparing EPC2T cells with or withoutNOTCH3knockdown. mRNA level for each gene in NS control cells was set to 1. *P< 0.05 vs. NS,n= 3.dSchematic ofNOTCH3second intron (N3Int2) region and ChIP PCR primers infand Supplementary Fig.4e. Primers amplify the region lacking ZEB1 or CSL-binding sites.eTransfection assays forpGL3-N3Int2-lucreporter activity with or without ectopic ZEB1 or ZEB2 expression.bla, empty vector control for ZEBs. *P< 0.05 vs.blaandpGL3-luc(empty reporter);#P< 0.05 vs.blaandpGL3-N3Int2-luc; ns not significant vs.blaandpGL3-N3Int2-luc;n= 4.fChIP assays for ZEB1 binding toN3Int2region in purified CD44L and CD44H cells. CD44L cells were stimulated with TGFβ for 14 days to induce CD44H cells. *P< 0.0005 vs. CD44L and IgG and TGFβ (−);#P< 0.005 vs. CD44H and IgG and TGFβ (−); **P< 0.05 vs. CD44L and anti-ZEB1 and TGFβ (+); ns not significant vs. IgG and TGFβ (−);n= 3.gRepresentative flow cytometry scatter plots of EPC2T cells withZEB1-targeted or NS control shRNA. *P< 0.05 vs. NS and TGFβ (−);#P< 0.0001 NS and TGFβ (+); ns not significant vs. NS and TGFβ (−);n= 3. Inb,g, flow cytometry was done 7 days following lentivirus infection. All bar diagrams represent mean ± s.d. At least three independent replicates were performed for all experiments. Fisher’s exact test was used for percentage comparisons ina. Student’st-test was used for paired data comparisons inb,c,f. ANOVA with Tukey’s post hoc test was used for multiple comparisons ine,g 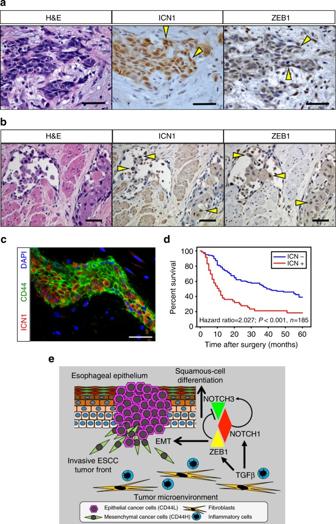Fig. 7 NOTCH1 activation and ZEB1 expression in invasive ESCC predicts poor prognosis.a,bRepresentative IHC images for ICN1 and ZEB1 in ESCC cells in a deep invasive tumor nest and ESCC cells invading into lymphatic vessels.aESCC #55;bESCC #62 in Supplementary Data1.cRepresentative IF image for ICN1 and CD44 in invasive ESCC cells. Scale bars, 50 μm ina–c.dSurvival curve for 185 post-surgical ESCC patients with or without ICN1 expression at the tumor invasive front.eModel of the role of Notch1 in EMT in ESCC. Notch1 activation promotes tumorigenicity and heterogeneity in SCC via EMT. Notch1 drives squamous-cell differentiation by inducing Notch3 in normal squamous epithelia as well as SCC cells. Notch3 limits EMT. In response to TGFβ from the tumor microenvironment (e.g., cancer-associated fibroblasts and inflammatory cells), however, transcriptional repression ofNotch3by ZEB1 permits Notch1-mediated induction of CD44H cells via EMT. Notch activation may result in the generation and maintenance of CD44H cells possessing mesenchymal properties and enhanced malignant potential. EMT allows neoplastic cells to cope with stress during carcinogenesis and disease progression (e.g., genotoxic stress induced by 4NQO). CD44H cells produce pro-tumorigenic cytokines (e.g., IL-6) and tissue remodeling factors (e.g., MMP13, LOX, and POSTN) (Supplementary Fig.3e) The ab27526 antibody recognizes a full-length NOTCH1 expressed on the cell surface in normal squamous epithelia [4] as well as well-differentiated SCC cells forming keratin pearl [11] . In this study, we have focused on cytoplasmic and nuclear intracellular Notch1 (ICN1) detected by anti-ICN1 V1744 . Transient transfection and dual-luciferase assays Transient transfection of reporter plasmids and luciferase assays was performed as described previously [4] , [80] . 1 × 10 5 cells were seeded per well in 24-well plates 24 h before transfection. Lipofectamine TM LTX and Plus TM reagents (Invitrogen) were used for DNA transfection, according to the manufacturer’s instructions. 400 ng of pGL3p-N3Int2 was transfected along with or without 400 ng of pBABE-bla-ZEB1, pBABE-bla-ZEB2 of pBABE-bla (empty vector control). 5 ng of phRL-SV40-renilla luciferase vector (Promega) was co-transfected to calibrate the variation of transfection efficiencies among wells. Cells were incubated in the presence or absence of 1 µg/ml DOX to induce ICN1 in cells expressing ICN1 TetOn for 48 h before cell lysis. Alternatively, 5 ng/ml TGFβ1 was added at 24 h after transfection and incubated for an additional 48 h before cell lysis. Luciferase activities were determined using Dual-Luciferase TM Reporter Assay system (Promega) and ORION Microplate Luminometer (Berthold Detection Systems, USA, Oak Ridge, TN). The mean of firefly luciferase activity was normalized with the co-transfected renilla luciferase activity. Transfection was carried out at least three times, and variation between experiments was not greater than 15%. ChIP assay 1 × 10 7 cells were treated with 1% formaldehyde for 10 min at 37 °C and quenched with 0.125 M glycine for 5 min at room temperature. Cross-linked chromatin was sheared into ~500 bp DNA fragments with Branson Sonifier 250 (Branson, Danbury, CT, USA) and subjected to immunoprecipitation with 2 µg/10 6 cells with antibody for ZEB1 (sc10572, Santa Cruz), NOTCH1 (sc6014-R, Santa Cruz) or either goat IgG (sc2028, Santa Cruz) or rabbit IgG (sc2027, Santa Cruz) as negative controls. DNA was purified by QIAquick PCR purification kit (QIAGEN, Valencia, CA) and analyzed by real-time PCR using StepOnePlus™ Real-Time PCR System (Applied Biosystems, Carlsbad, CA). The following primers were used for real-time qPCR: 5′-CCCACAGCCCAACTCGGAGG-3′ and 5′-CCGCGCCTGGAATACTGCCG-3′ for ZEB1-binding sites at the 2nd intron of NOTCH3 , 5′-GCTGGGCGCCGAGGATAG-3′ and 5′-AGACCTCGTCCCCATCTCCTAGTC-3′ for CSL-binding sites [4] at the 2nd intron of NOTCH3 , 5′-TGCCAAAAGAGGAAGCATAAGTA-3′ and 5′-TCAAAATCCCTGTGTAGCTGAAT-3′ for an off-target control [4] for NOTCHotch3 . 5′-CCCTTTCTGATCCCAGGTCT-3′ and 5′-GACCTGCACGGTTCTGATTC-3′ for a ZEB1-binding site on the of CDH1 promoter [87] , 5′-GAAGTGGCTCCAGTGCTCAAA-3′ and 5′-ATGGCAGTGCATGCCTGTAGT-3′ for an off target control for CDH1 promoter [87] , 5′-CGTGTCTCCTCCTCCCATT-3′ and 5′-CCGCTGTTATCAGCACCAG-3′ for a CSL-binding site at the HES1 promoter [88] , 5′-TGGATCCAATCCTATTGCCC-3′ and 5′-CGCAGCAGTTGGAAGTGTTT-3′ for an off target control for HES1 [88] . Data represent three independent experiments. Statistical analyses Data from experiments were presented as mean ± standard error ( n = 3–6) in real-time RT-PCR, luciferase assays, flow cytometry and IHC labeling index or mean ± standard deviation ( n = 8–12) in xenograft transplantation tumor analyses. GraphPad Prism 7 (GraphPad Software, La Jolla, CA) or Stata Version 14 (StataCorp, College Station, TX) software were used for statistical analyses. The two-tailed Student’s t- test was used for paired comparisons. Fisher’s exact test was used for percentage comparisons in xenograft experiments. ANOVA with Tukey’s post hoc test was used for multiple pairwise comparisons. P < 0.05 was considered significant. The Kappa Statistic was used to evaluate concordance between NOTCH1-positive IHC staining as classified by independent antibodies. Survival curves were estimated using the Kaplan–Meier method and plotted. Candidate predictor variables were tested at P < 0.05 by univariate and multivariate Cox Regression using the z -score corresponding to the hazard ratio. Data availability Microarray data were deposited at the NCBI Gene Expression Omnibus ( http://www.ncbi.nlm.nih.gov/geo ) under accession number GSE37994. All data sets are available from the authors upon request.